A metabolic view on menopause and ageing The ageing of the global population calls for a better understanding of age-related metabolic consequences. Here we report the effects of age, sex and menopause on serum metabolites in 26,065 individuals of Northern European ancestry. Age-specific metabolic fingerprints differ significantly by gender and, in females, a substantial atherogenic shift overlapping the time of menopausal transition is observed. In meta-analysis of 10,083 women, menopause status associates with amino acids glutamine, tyrosine and isoleucine, along with serum cholesterol measures and atherogenic lipoproteins. Among 3,204 women aged 40–55 years, menopause status associates additionally with glycine and total, monounsaturated, and omega-7 and -9 fatty acids. Our findings suggest that, in addition to lipid alterations, menopause may contribute to future metabolic and cardiovascular risk via influencing amino-acid concentrations, adding to the growing evidence of the importance of amino acids in metabolic disease progression. These observations shed light on the metabolic consequences of ageing, gender and menopause at the population level. With global population aging we are facing substantial social, economic and health-care issues. Aging relates closely to a wide spectrum of metabolic and other chronic diseases. The disease burden significantly differs by age and sex. Menopause is an endocrinological transition strongly influencing health and disease susceptibility of all middle-aged and elderly women. It is defined as the permanent cessation of menstruation resulting from the loss of ovarian follicles. Menopause is preceded by menopausal transition, a period of menstrual cycle irregularity, which usually begins in the mid 40s. Menopause is not a distinct event at a discrete point in time but rather a continuous dynamic process of progressive decline in ovarian function and circulating oestrogen levels, with substantial interpersonal age-of-onset variation. Menopause has substantial health consequences ranging from disturbances in lipid and glucose metabolism to psychological stress and sleep alterations [1] , [2] . Importantly, menopause is closely linked with cardiovascular diseases (CVDs), the leading cause of death worldwide, although the significance of menopause as a CVD risk factor has been challenged [3] , [4] , [5] , [6] . Premenopausal women have lower CVD incidence and mortality rates compared with men of the same age, which is partly explained by the protective effects of endogenous oestrogens against atherosclerosis [7] , [8] . Loss of ovarian function during natural or artificial menopause and subsequent hypoestrogenism is believed to promote CVD. Large cohort studies have firmly established increased CVD risk after bilateral oophorectomy, causing sudden menopause [9] , [10] . Early menopause may have a modest effect on CVD risk [11] ; however overall, the relationship between postmenopausal status and CVD remains somewhat unclear. Menopause nevertheless influences several CVD risk factors, and some menopausal symptoms, such as the prevalence of vasomotor episodes, may reflect CVD susceptibility [12] . Earlier studies reported lower high-density lipoprotein cholesterol (HDL) concentration [6] combined with higher low-density lipoprotein cholesterol (LDL) [6] , triglycerides (TGs) and total cholesterol (TC) concentrations [13] among postmenopausal women compared with age-matched premenopausal controls. Later reports suggested LDL cholesterol and apolipoprotein-B (apoB) as age-independent menopausal biomarkers, whereas results on TC, HDL and TG have been controversial [14] , [15] . HDL tends to lose its protective effects against CVD after menopause, with an atherogenic shift to higher HDL particle number and smaller HDL particle size [16] . A recent study suggests an alternative hypothesis, namely that an increased premenopausal cardiovascular risk profile, with higher TC, blood pressure and overweight, promotes by itself early menopause [17] . Studies utilizing modern metabolomic approaches have recently proposed novel biomarkers for future insulin resistance [18] , type II diabetes (T2D) [19] , CVD [20] and mortality [21] . Metabolome-wide gender [22] and age [23] issues have been previously assessed as separate entities. We aimed to simultaneously investigate the influence of age and gender on serum metabolites, further including a key player behind gender differences: menopause. We present data on 26,065 individuals of Northern European ancestry from Finland and Estonia. Assessing a wide spectrum of 135 metabolite measures with highly detailed lipid components sets the scope of metabolomic profiling far beyond the traditional laboratory measures and helps to detect minor changes in metabolically important parameters at the individual level. Our results highlight the differences in metabolite fingerprints by gender and show that menopause raises the levels of several lipoprotein and lipid measures and, interestingly, also the levels of amino-acid measures. Study setting We analysed the effects of age and menopause on systemic metabolomics in altogether 16,107 Finnish and 9,958 Estonian individuals (8,321 and 6,416 women, respectively). 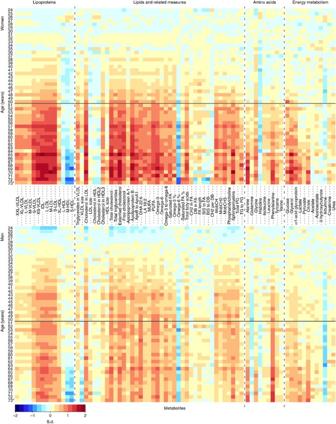Figure 1: Heat maps demonstrating age-related changes in the metabolites in 3,009 FINRISK-97 women (upper panel) and 3,450 men (lower panel). One-year age groups are displayed on theyaxis and individual metabolites on thexaxis. Colours represent the divergence in units of s.d. from the mean of the metabolite levels of 24–35 year olds. Heat maps of the Estonian cohort are presented in theSupplementary Fig. 3. The horizontal lines are set at the mean age of menopause, 51 years. Lipoprotein subclasses represent particle concentration of each subclass. VLDL=very low-density lipoprotein, IDL=intermediate-density lipoprotein, LDL=low-density lipoprotein, HDL=high-density lipoprotein, ApoB=apolipoprotein-B, ApoA-1=apolipoprotein A-1, DHA=docohexanoid acid, LA=linoleic acid, MUFA=monounsaturated fatty acids, PUFA=other polyunsaturated fatty acids than 18:2, FA=fatty acids, CH2=methylene groups, DB=double bonds, BIS=bisallylic groups, MobCH=double bond protons of mobile lipids, MobCH2=CH2 groups of mobile lipids, MobCH3=CH3 groups of mobile lipids, PG=phosphoglycerides, TG=triglycerides. The study comprises seven independent Finnish cohorts and a large population cohort from Estonia (EGCUT, Table 1 ). Individuals using lipid-lowering medication, having diabetes or being pregnant were excluded from all analyses, and individuals using hormone replacement therapy (HRT) were additionally excluded from menopause analyses ( Table 1 ). The metabolites were produced from serum (Finnish) or plasma (Estonian) samples using nuclear magnetic resonance (NMR)-based methods [24] , [25] , including well-defined lipid components. The 135 metabolites analysed include 74 lipoprotein, 17 lipid and 23 fatty acid-related measures, accompanied by 9 amino acids and 12 small molecules related to cell energy metabolism ( Supplementary Table 1 ). The Estonian samples lacked information on some lipid and fatty acid components ( Supplementary Table 1 ). Menopause status was defined based on questionnaire data. In addition, follicle-stimulating hormone measures were available in the Finnish cohort DILGOM; the questionnaire data highly correlated with hormone measures in dissecting the menopausal status. All the participants gave written informed consents, and the study cohorts have local ethical board approvals. Table 1 Characteristics of the study cohorts. Full size table A correlation matrix revealed significant metabolite–metabolite correlations among the 135 metabolites ( Supplementary Fig. 1 ). Principal component (PC) analysis showed altogether 22 PCs explaining >95% of the variation seen in the data set ( Supplementary Data 1 ). The multiple testing corrected significance level in the highly correlated data was set accordingly ( P <0.05/22 PCs, that is, P <0.0023). Further, based on high correlation, only the total particle concentration of each lipoprotein subclass was used in the analyses. Detailed lipid profiles differ by age and gender To explore age–metabolite relations, we constructed a heat map ( Fig. 1 ) of the largest Finnish cohort, FINRISK-97 ( n =8,444, age range 24–75 years). For each metabolite, the divergence (in units of s.d.) from the mean level of those younger than 35 years was plotted for each 1-year age group. The reference group was chosen to represent a generally healthy population rarely having age-related metabolic disorders. As previous studies have suggested gender differences in the metabolite profiles [22] , a gender-specific approach was chosen. The heat maps revealed clear age–sex-related metabolomic fingerprints: among men ( Fig. 1 ; Supplementary Fig. 2a,b ), lipoprotein measures of very low-density lipoprotein cholesterol (VLDL), intermediate-density lipoprotein cholesterol (IDL) and LDL, as well as serum total, free and esterified cholesterol, serum TG and apoB all increased starting from the early 30s. The amount of larger HDL particles increased by age, whereas the measures associated with medium and small HDL declined, except for TG in small HDL, which increased. Several metabolites expressed non-linear behaviour by age; this was most evident for the VLDL measures having a parabolic age relation first increasing but later declining among the oldest men. Figure 1: Heat maps demonstrating age-related changes in the metabolites in 3,009 FINRISK-97 women (upper panel) and 3,450 men (lower panel). One-year age groups are displayed on the y axis and individual metabolites on the x axis. Colours represent the divergence in units of s.d. from the mean of the metabolite levels of 24–35 year olds. Heat maps of the Estonian cohort are presented in the Supplementary Fig. 3 . The horizontal lines are set at the mean age of menopause, 51 years. Lipoprotein subclasses represent particle concentration of each subclass. VLDL=very low-density lipoprotein, IDL=intermediate-density lipoprotein, LDL=low-density lipoprotein, HDL=high-density lipoprotein, ApoB=apolipoprotein-B, ApoA-1=apolipoprotein A-1, DHA=docohexanoid acid, LA=linoleic acid, MUFA=monounsaturated fatty acids, PUFA=other polyunsaturated fatty acids than 18:2, FA=fatty acids, CH2=methylene groups, DB=double bonds, BIS=bisallylic groups, MobCH=double bond protons of mobile lipids, MobCH2=CH2 groups of mobile lipids, MobCH3=CH3 groups of mobile lipids, PG=phosphoglycerides, TG=triglycerides. Full size image The female metabolomic fingerprint ( Fig. 1 ; Supplementary Fig. 2c,d ) significantly differed from the male one. The concentrations of the atherogenic metabolites were relatively stable until a rapid increase occurred at the age of late 40s and early 50s, stabilizing thereafter. Similar to men, VLDL, IDL and LDL concentrations, serum cholesterol measures, larger HDL measures and TG in small HDL all increased by age, and medium and small HDLs declined in the FINRISK-97 women. The age–sex-related patterns in lipids and lipoproteins seen in FINRISK-97 were tested for replication in the Estonian EGCUT cohort ( n =9,958, age range 18–103 years). Inspection of the male EGCUT heat map ( Supplementary Fig. 3a ) showed a similar shift towards atherogenicity in the lipid metabolites as detected among the Finnish men; however, the timing for this change was earlier starting already at the age of 27 years. Especially the VLDL measures expressed a steeper U-shape. Among the Estonian women, again a clear change towards a more atherogenic lipid profile occurred between 45 and 50 years of age ( Supplementary Fig. 3b ). Age–sex interaction analysis in 40- to 55-year-old participants The heat maps indicated a major change in the female metabolic fingerprint timing between 45 and 50 years of age, which clearly overlaps the period of menopausal transition. To evaluate the heat map observations, we assessed the gender–age effects on metabolites during the menopausal transition period (40–55 years, n =3,478) in random effects meta-analysis of three Finnish cohorts (FINRISK-97, DILGOM and Health2000, containing participants in this age group). We fitted a linear model including an age × sex interaction term, further adjusted for body mass index (BMI), daily smoking status and fasting time before sampling. 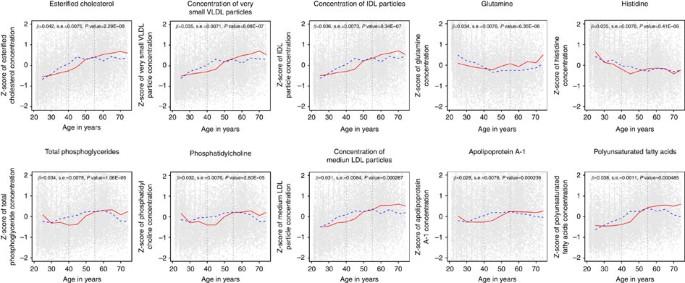Figure 2: Illustration of the key menopause-associating metabolite concentrations by age fit with natural cubic splines. Altogether, 6,790 Finnish men (blue line) and 7,544 women (red line) were analysed with natural splines, utilizing univariate regression, using z-standardized values (individual values subtracted from the mean and divided by s.d.). Knots are placed at every 5 years. Standardization was performed separately in men and women; thus, the absolute values are not comparable between sexes.Pvalues outline age × sex interaction effects on the metabolite concentrations, calculated using multivariate liner regression in random effects meta-analysis (see alsoTable 2). Significant age–sex interactions were observed with 10 metabolites ( Table 2 ). Oesterified cholesterol showed the strongest interaction, followed by lipoprotein particle concentrations of very small VLDL, IDL and medium LDL, total phosphoglycerides, phosphatidylcholine and apolipoprotein A-1 (apoA-1), amino acids glutamine and histidine, and polyunsaturated fatty acids (PUFAs). Figure 2 demonstrates the age–sex relations by natural cubic splines, calculated using all the Finnish data (7,786 men and 8,321 women), of the 10 metabolites with significant age–sex interactions, showing the general trend of atherogenic lipoprotein and lipid concentrations increasing and reaching the steady state around the age of 30 years in males and a sudden change around the age of 45 in females. The rest of the VLDL and LDL subclass particle concentration and several fatty acid concentrations (omega-6, omega-7 and -9 and saturated fatty acids, linoleid acid, docosahexanoid acid, monounsaturated fatty acid (MUFA) and total fatty acids) followed a similar pattern but did not reach the multiple testing corrected significance level of P <0.0023 ( Supplementary Fig. 4 ; Supplementary Table 2 ). On the other hand, only minor differences in sex-specific profiles were detected in the HDL measures ( Supplementary Fig. 4 ; Supplementary Table 2 ). Table 2 Age–sex interaction on metabolite levels in random effects meta-analysis among 40- to 55-year-old Finnish men and women. Full size table Figure 2: Illustration of the key menopause-associating metabolite concentrations by age fit with natural cubic splines. Altogether, 6,790 Finnish men (blue line) and 7,544 women (red line) were analysed with natural splines, utilizing univariate regression, using z-standardized values (individual values subtracted from the mean and divided by s.d.). Knots are placed at every 5 years. Standardization was performed separately in men and women; thus, the absolute values are not comparable between sexes. P values outline age × sex interaction effects on the metabolite concentrations, calculated using multivariate liner regression in random effects meta-analysis (see also Table 2 ). Full size image Assessing menopausal effects We further assessed the impact of menopause status on the metabolite levels in a random effects meta-analysis in female participants of all age groups. Altogether 10,083 Finnish and Estonian women were included in the analysis. 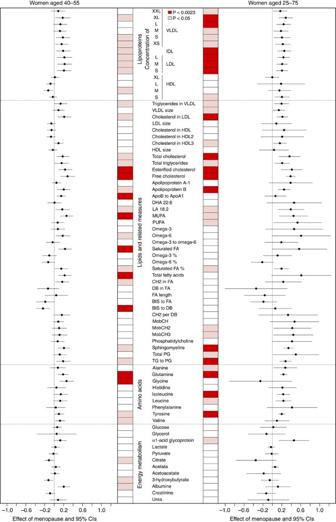Figure 3: The association of the metabolites with menopause status in Finnish and Estonian women in random effects meta-analysis using multivariate linear regression. The effect sizes and 95% confidence intervals are presented. Values from linear regression model are adjusted for age, BMI, smoking and time of fasting before sampling. On the left side, results of the women in the menopausal transition window (aged 40–55 years,n=3,204), and results of all women (21–75 years,n=10,083) on the right side of the figure. Dark-red colour indicates aPvalue below the Bonferroni corrected significance level (P<0.0023), whereas light-red colour indicatesP<0.05.βindicates the effect size in s.d. within the rank-normalized values. VLDL=very low-density lipoprotein, IDL=intermediate-density lipoprotein, LDL=low-density lipoprotein, HDL=high-density lipoprotein, ApoB=apolipoprotein-B, ApoA-1=apolipoprotein A-1, DHA=docohexanoid acid, LA=linoleic acid, MUFA=monounsaturated fatty acids, PUFA=other polyunsaturated fatty acids than 18:2, FA=fatty acids, CH2=methylene groups, DB=double bonds, BIS=bisallylic groups, MobCH=double bond protons of mobile lipids, MobCH2=CH2 groups of mobile lipids, MobCH3=CH3 groups of mobile lipids, PG=phosphoglycerides, TG=triglycerides. The results are presented in Table 3 and Fig. 3 . Postmenopausal women had significantly higher concentrations of serum total, esterified and free cholesterol, apoB, very large and large VLDL particles, all the LDL particle subclasses and IDL particles, and TC in LDL compared with premenopausal women ( Table 3A ; Fig. 3 ). Postmenopausal women also had significantly higher concentrations of amino acids glutamine, tyrosine and isoleucine, as well as sphingomyelins and the ratio of TG to phosphoglycerides ( Table 3A ; Fig. 3 ). Potential cohort-induced variability was estimated with the I 2 measure of heterogeneity. The mean I 2 for the HDL measures was 86.1, for VLDL measures 63.0, for LDL measures 68.2 and for fatty acids and related measures 87.1. The amino acids glutamine, tyrosine and isoleucine all had relatively low between-cohort variability ( I 2 <35), whereas greater heterogeneity was seen with glycine, valine and isoleucine ( I 2 >80). Table 3 The association of the metabolites with menopause status in random effects meta-analysis using ultivariate linear regression in (a) 21- to 75-year old ( n =10,083) and (b) 40- to 55-year-old ( n =3,240) Finnish and Estonian women. Full size table Figure 3: The association of the metabolites with menopause status in Finnish and Estonian women in random effects meta-analysis using multivariate linear regression. The effect sizes and 95% confidence intervals are presented. Values from linear regression model are adjusted for age, BMI, smoking and time of fasting before sampling. On the left side, results of the women in the menopausal transition window (aged 40–55 years, n =3,204), and results of all women (21–75 years, n =10,083) on the right side of the figure. Dark-red colour indicates a P value below the Bonferroni corrected significance level ( P <0.0023), whereas light-red colour indicates P <0.05. β indicates the effect size in s.d. within the rank-normalized values. VLDL=very low-density lipoprotein, IDL=intermediate-density lipoprotein, LDL=low-density lipoprotein, HDL=high-density lipoprotein, ApoB=apolipoprotein-B, ApoA-1=apolipoprotein A-1, DHA=docohexanoid acid, LA=linoleic acid, MUFA=monounsaturated fatty acids, PUFA=other polyunsaturated fatty acids than 18:2, FA=fatty acids, CH2=methylene groups, DB=double bonds, BIS=bisallylic groups, MobCH=double bond protons of mobile lipids, MobCH2=CH2 groups of mobile lipids, MobCH3=CH3 groups of mobile lipids, PG=phosphoglycerides, TG=triglycerides. Full size image We then targeted the model to those women in the menopausal transition window (aged 40–55 years, n =3,240), to better focus on the effects of menopause as opposed to ageing. Postmenopausal women had significantly higher concentrations of amino acids glutamine and glycine, whereas suggestive association was seen with tyrosine and valine ( Table 3B ; Fig. 3 ). Postmenopausal women also had significantly higher concentrations of MUFA, total and omega-7 and -9 fatty acids ( Table 3B ; Fig. 3 ). In addition, significant menopausal associations were seen with free and esterified cholesterol and the apoB/apoA-1 ratio ( Table 3B ; Fig. 3 ). Postmenopausal women had less bisallylic groups per double bond than premenopausal women. The lipoprotein subclass concentrations showed a similar trend as among all women; however, the results did not reach statistical significance ( Fig. 3 ; Supplementary Table 3 ). The HDL measures (mean I 2 =2.7), fatty acids and related measures (mean I 2 =10.5), and amino acids glutamine, tyrosine, isoleucine and valine ( I 2 <27) had relatively low cohort variability, whereas mean I 2 for LDL measures was 37.1 and for VLDL measures 44.0. Sensitivity analyses As all women using HRT were excluded from the analyses because of uncertain menopausal status, we performed a sensitivity analysis on possible HRT effects on metabolomic fingerprint. Finnish 40- to 60-year-old HRT users ( n =1,053) were compared with premenopausal non-users ( n =813) and separately with postmenopausal non-users ( n =735) of the same age group in random effects meta-analysis ( Supplementary Table 4 ). The metabolomic profile of HRT users did not differ significantly from the premenopausal non-users with any of the metabolites, whereas the postmenopausal non-users had pro-atherogenic changes in their lipid profile compared with the HRT users in terms of higher values of ApoB and ApoB/ApoA-1 ratio, and higher concentration of very small and very large VLDL particles, large LDL particles and IDL particles, and lower concentrations of large HDL particles, lower TC in HDL and HDL 2 , as well as smaller diameter of HDL particles. Postmenopausal non-users also had higher values of albumin and glycoprotein acetyls than the HRT users. Sensitivity analyses were also performed to assess potential impacts of fasting time variability as well as age effects. Random effects meta-analysis among Finnish 40- to 55-year-old women ( n =1,804) revealed significant age effects with several metabolites, including amino acids, lipids and lipoproteins ( Supplementary Table 5 ). Fasting time was assessed accordingly ( n =1,490); however, significant influence was seen only with four metabolites ( Supplementary Table 6 ). The HDL measures, measures describing fatty acid saturation and measures of small molecules related to cell energy metabolism did not show consistent association with menopause status or an age–sex interaction ( Supplementary Tables 2 and 3 ). The concentrations of TC in HDL, HDL 2 and HDL 3 particles also remained relatively stable despite ageing, whereas small and medium HDL concentrations declined by age in both sexes, and very large HDL increased ( Supplementary Fig. 4 ). We assessed the effects of age, sex and menopause on metabolites among >26,000 Finnish and Estonian participants of Northern European ancestry. The study provides examples of gender-specific metabolic fingerprints at the population level, showing association of menopause with cholesterol components, amino acid and fatty acid concentrations, and an evident pattern of pro-atherogenic lipid changes. Among men, the concentrations of these lipid measures rise already at early middle age. Premenopausal women have significantly lower mean values until a rapid increase around the age of 45, where the atherogenic lipid concentrations suddenly bounce, bypassing the mean values of men. This pattern is consistent for all the cholesterol measures analysed, all the VLDL, IDL and LDL subclass particle concentrations, as well as for TG measures and apoB. Menopause-associated oestrogen depletion has several well-established metabolic consequences. Menopause promotes atherosclerosis through changes in lipid profile, endothelial dysfunction and oxidative stress [26] , [27] . Hormonal changes in menopause promote higher body fat, in particular abdominal obesity, contributing to the increased CVD and metabolic risk [28] , [29] . Hormone levels do not, however, independently predict dyslipidemias or CVD events [30] . Menopause is most likely one of the key players behind the substantial differences observed here between the male and female age-specific metabolic fingerprints. High TC, LDL, TG and apoB values have also previously been associated with menopause [14] , [15] , [29] , [31] . These lipid disturbances may be especially harmful in hyperglycaemic environment promoting oxidative injury [31] , [32] . Recent studies have targeted to more detailed lipid profiles, beyond the traditional measures of TC, total LDL cholesterol or TG. Menopause may affect the concentrations of small, dense LDL alone and with apoB [33] . VLDL size and IDL particle number have been proposed as predictors for stroke in postmenopausal women [34] , and both small, dense LDL and small-sized HDL have displayed predictive value for future T2D in women [32] . Our results provide insights into highly detailed lipid subclass measures by age and sex in a population free of diabetes and not using lipid-lowering medication. We observed significant associations of free and esterified cholesterol and the apoB/apoA-1 ratio with menopause status among 40- to 55-year-old women, postmenopausal women having significantly higher values. Esterified cholesterol, very small VLDL, IDL, medium LDL and apoA-1 were among the key findings in the age–sex interaction analysis, suggesting a significant gender influence on these measures. These findings also highlight the role of menopause as a CVD risk factor. Via pro-atherogenic lipid alterations menopause significantly contributes to CVD risk. Phosphoglycerides, sphingomyelins and phosphatidylcholine and other cholines, all related to lipoprotein assembly, also showed significant age–sex interaction or association with menopause status. The menopause-induced increase in these lipoproteins, lipids and fatty acids likely reflects the influence of hormonal alterations on liver enzymes [35] , [36] but might also relate to weight gain and insulin resistance [37] , [38] . The HDL measures analysed did not show consistent association with menopause or an age–sex interaction, being in line with the emerging understanding of absolute HDL concentration being a poor indicator of HDL functional capacity [39] . The relation of obesity, insulin secretion and branched-chain amino acids has been studied for decades [40] . Recently, branched-chain and aromatic amino acids, leucine, isoleucine, valine, tyrosine and phenylalanine have been linked to insulin resistance [17] and risk of future T2D [18] , some in an obesity-dependent manner [17] . A risk score of amino acids tyrosine, phenylalanine and isoleucine has been shown to predict future T2D [19] and CVD [20] in healthy individuals. Glutamine and glutamic acid metabolism may contribute to the regulation of glucose metabolism and insulin secretion in diabetic patients in a protective manner [41] , [42] , [43] . High glutamine-to-glutamate ratio reduced the risk of incident diabetes in mice [44] . On the other hand, parenterally or enterally administrated glutamine is suggested to have cardioprotective effects in patients undergoing cardiac surgery [45] , [46] . Qi et al. [47] have recently established a novel risk locus for coronary heart disease among diabetic patients, located in the GLUL gene. The mechanisms by which alterations in the metabolism or concentration of glutamine, glutamate or their precursors may increase CVD risk are unclear. At the population level in humans, metabolomics profiling with mass-spectrometry data has linked several amino acids, including glutamine and isoleucine, with glucose intolerance and T2D [48] , and glutamine concentration, has been positively associated with higher intimamedia thickness of carotid artery as well as with coronary artery atherosclerosis [49] . The same study also linked tyrosine concentrations with these two CVD-related end points. Here postmenopausal women had higher glutamine, tyrosine and isoleucine concentrations than premenopausal women, suggesting a role for menopause in their regulation. Among 40–55-year-old women, the values of glutamine and glycine were significantly higher in postmenopausal than in premenopausal women, and tyrosine and valine showed suggestive associations. Menopause may thus contribute to the risk of cardiometabolic end points by affecting amino-acid levels, in addition to lipid alterations and obesity. The associations of amino-acid concentrations with menopause have not been previously reported in large population samples. Fatty acid composition and intake modulate CVD risk in several ways. Omega-3 PUFAs act cardioprotectively via anti-inflammatory and blood pressure-lowering actions [50] . Higher PUFA intake is associated with lower CVD incidence and mortality [51] , [52] . Docosahexaenoic acid, belonging to omega-3 long-chain PUFA, is proposed to have TG-lowering capacity [53] . Trans -fatty acid concentrations [54] and high intake [51] are linked with increased CVD risk, whereas long-chain MUFA are linked with the risk of congestive heart failure [55] . Menopause affects fatty acid metabolism at least through obesity-related changes and altering tissue fatty acid metabolism. Oestrogen affects tissue PUFA content [56] and the capacity of adipose tissue to uptake and store fatty acids in TG-enriched lipid droplets [57] . In postmenopausal women, PUFA intake improved endothelial function [27] and physical performance [58] . Fatty acids also play a role in ageing; small-to-medium-chain saturated fatty acids were inversely associated with telomere length in postmenopausal women in a recent study [59] . Our observations with MUFA, total and omega-7 and -9 fatty acids associating with menopause status and significant age–sex interaction seen with PUFA contribute to the current understanding of the menopausal influence on CVD-related pathways. The same trend in age–sex interactions was also seen with several other fatty acids (omega-6, omega-7 and -9 fatty acids, docosahexaenoid acid, and linoleic acid). Unfortunately, nutritional data on fatty acid intake were not available to assess the role of diet in the observed menopausal associations. A thorough assessment of premenopause, perimenopause and menopause would require highly detailed targeting of the final menstrual period and the appearance of the preceding menopause-related symptoms, including longitudinal hormone and risk factor measures before, during and after the menopausal transition [60] . The vast majority of large population studies lack such information, relying on questionnaire data and being cross-sectional in nature. Factors such as surgical menopause and the wide use of HRT and other hormonal agents masking the postmenopausal hallmarks further blur the recognition of natural menopause. In addition, menopause-related hormonal alterations and hence the potential menopausal effects on, for example, CVD risk factors begin already years before the final menstrual period or any notable symptoms [61] . We verified the questionnaire-based menopausal data were partly using hormone measurements, and the two were very well in line with each other. Reliable recognition of perimenopausal women was however impossible, and all the women using HRT were excluded as menopause status was analysed as a dichotomous end point. A sensitivity analysis comparing HRT users with pre- and postmenopausal non-users suggested that the metabolomic profile of the HRT users resembled that of premenopausal women, whereas the postmenopausal non-users had pro-atherogenic changes in their lipid profile compared with the HRT users. The importance of menopause as a CVD risk factor is controversial. While artificial menopause by bilateral oophorectomy has been associated with increased CVD risk [9] , [10] , large cohort studies have failed to establish the link between menopause and CVD [3] , [4] , [5] , [6] . Menopause does, however, influence several CVD risk factors. Our results link menopause with amino-acid alterations, which in turn have been linked with CVD [20] , insulin resistance [17] and T2D [18] , [19] , [20] in separate, large population studies. Individual lipid markers such as LDL and HDL cholesterol have been shown to predict CVD since the 1950s, and menopause influences these lipid traits in a pro-atherogenic manner [14] , [15] , [16] . Here menopause had a pro-atherogenic influence on several lipids and lipoprotein subclasses. Postmenopausal women not using HRT also had signs of pro-atherogenic lipid profile compared with the HRT users. These findings elucidate the potential impact of menopause in cardiometabolic processes. A major strength of this study is the substantial sample size of over 26,000 participants. The metabolites were measured in the same laboratory. Limitations of this work include the cross-sectional design, allowing crude estimates of menopausal status. Assessment of menopause as a continuous variable ranging from premenopause to perimenopause to late postmenopause, more closely reflecting the underlying biology, was however beyond the reach of the questionnaire data. Age of the participants varied from 21 to 103 years. Heat maps, used to assess the age effects, revealed significant age effects on several metabolites, which were also detected in sensitivity analysis. Nevertheless, menopause status still had a significant impact on several metabolites. In FINRISK-97, DILGOM and EGCUT cohorts, only semi-fasting state was required before sampling. Although all analyses were corrected for age and fasting time, variances between the cohorts analyzed may have an impact on the results. The potential cohort-induced variation was controlled for using meta-analysis-based methods. The heterogeneity seen in random effects meta-analysis may hint on age or sex influence, or reflect differences in fasting time. Relatively low between-cohort variance was seen with amino acids glutamine, isoleucine and tyrosine, and these amino acids may be less sensitive to age and sex effects than amino acids glycine, valine and phenylalanine. The same cohorts have been utilized in a similar study setting previously [21] , [25] , [62] . The study comprised individuals of Northern European ancestry, and the findings may vary in other populations. Nutritional data on fatty acid intake were not available to evaluate the potential nutritional influence on menopause-related findings. Metabolites were analysed from serum samples in all the Finnish study cohorts, but from plasma in the Estonian study sample, which may produce some variability across the cohorts, although the correlation between serum- and plasma-based values has been reported to be high for the majority of the metabolites [63] . Serum metabolome comprises thousands of components related to systemic metabolism, of which NMR-based applications only capture a small fraction. Nevertheless, NMR makes metabolomics available for the masses and has facilitated a variety of novel scientific findings. Currently, NMR-based applications are the only approaches that can offer fully automated and highly reproducible high-throughput experimentation in a very cost-effective manner [64] . Cost effectiveness via high-throughput, along with absolute quantification of molecular measures, is a prerequisite for metabolomics methodologies in epidemiology. Further associations of menopause-induced metabolite alterations with diagnostic disease end points, such as CVD or T2D, should be evaluated in future studies, thus widening the biological relevance of the results presented here. Despite these limitations, our findings unravel age and menopausal effects on serum metabolome, adding to the current understanding of menopause-induced metabolic changes. To summarize, our results demonstrate that metabolic fingerprints are strongly age- and sex-dependent. Men enter the pro-atherogenic phase already in the early middle age. In women, a clear atherogenic shift overlapping the menopausal transition is observed. Our findings of a menopause-specific increase regarding several amino acids and fatty acids suggest a menopausal influence on numerous pathways contributing to the pathogenesis of diabetes and of CVDs. Study cohorts This study comprises seven independent Finnish study cohorts and an Estonian population sample, totalling 26,065 individuals ( Table 1 ). All the study cohorts have been previously described in detail [65] , [66] , [67] , [68] . FINRISK cohort samples are collected every 5 years in five separate geographical areas in Finland. In each survey 8,000–10,000 persons aged 24–75 years are invited to fill in questionnaires and to participate in a clinical examination and blood tests. The FINRISK-97 sample was collected in 1997 and had 8,444 participants. The DILGOM sample is a subset of the FINRISK-07 collection with 555 individuals from the Helsinki region examined in great detail for metabolic risk factors. Health2000 is an independent study sample with 8,223 participants from Finland. Metabolome data were available for 1,364 participants belonging to a subset with detailed CVD risk factor measures, all ≥45 years. The Young Finns (YF) study assesses CVD risk factors among 3,500 young individuals, who at baseline were 3–18 years of age. Serum samples for the metabolomics analyses were drawn in 2001, when participants were 24–39 years of age. Helsinki Birth Cohort Study (HBCS) comprises participants born in 1934–1944 in Helsinki, Finland. In HBCS, metabolome data was available for 853 individuals. FinnTwin16 (FT16) is a longitudinal twin cohort study with 5,563 Finnish twins born 1974–1979. FinnTwin12 (FT12) sample consists of 5,362 Finnish twins born in 1983–1987 followed longitudinally. Metabolome data were available for 554 and 776 participants, respectively, collected during a clinical study in young adulthood. The EGCUT sample is an Estonian population cohort with metabolome data of 9,958 participants aged 18–103 years. All cohorts have detailed questionnaire data with medical examination at the time of metabolome serum sampling. All participants gave written informed consent, and all studies have local ethical committee approvals (the ethics committee of Finnish National Health Institute for FINRISK-97 (38/96) and Health2000 (407/E3/2000), the ethics committee of Helsinki University Hospital, Finland (IRB00003181), for DILGOM (229/E0/2006), the twin cohorts (346/E0/05 and 113/E3/2001) and HBCS (334/E3/2000), the 1st ethical committee of Southwestern Hospital District, Finland, for the YF study (3/2000), and the ethics committee of the University of Tartu, Estonia, for EGCUT (205/T-20). Serum metabolites The same high-throughput 1 H NMR metabolomics platform in the same laboratory was used to produce all the metabolite variables used in the study, including the Estonian ones. The method has been described in detail elsewhere [24] , [25] , [62] . The NMR-based metabolome technique yields data on 135 serum metabolites and ratios ( Supplementary Table 1 ). These include 74 lipoprotein subclass measures, 17 lipid measures, 23 fatty acids and measures related to fatty acid saturation, 9 amino acids and 12 small molecules, many involved in cell energy metabolism. The metabolites were produced from serum in all the Finns and from plasma in Estonians. Assessing menopause Menopausal status was assessed first by defining participants aged 35 or younger as premenopausal and those aged 56 years or more as postmenopausal, unless otherwise stated in the questionnaire, for example, due to surgical menopause. Questionnaire data were then used to distinguish the menopause status for the remaining individuals. All women <55 years reporting regular menstruation without hormonal agents were classified as premenopausal, and all women >35 years reporting having their final menstrual period more than 1 year ago were stated postmenopausal, together with all women who had undergone surgical menopause. HRT users and participants with missing or incomprehensive menstrual data were excluded due to uncertain menopausal status ( n =1,202). Hormone measures or longitudinal data on menstruation were not available. In addition, we excluded pregnant women and those men and women using diabetes medication or statins in order to control for confounding factors ( n =1,248 in total). Follicle-stimulating hormone measures from serum (S-FSH, IU l −1 ) were available for 271 women in the DILGOM study cohort and were used to verify the questionnaire data. Postmenopausality limit of S-FSH ≥26 IU l −1 , recommended by the Helsinki University Central Hospital laboratory, was utilized. The correlation of the questionnaire results and hormone-based menopausal approximation was extremely high: only three women were determined postmenopausal according to the questionnaire but had S-FSH <15 IU l −1 each, and two women classified as premenopausal had S-FSH>26 IU l −1 . Statistical analyses R (version 2.12 or higher, http://www.r-project.org/ ) was used for all statistical analysis. Correlation matrix and PCs Pairwise Spearman’s rank correlation coefficients were calculated from the metabolite concentrations of the combined data set of the Finnish cohorts ( n =12,629) with the cor.test function (method=’spearman’) and plotted with the heat map.2 function in the gplots package of R. The correlation matrix is presented in Supplementary Fig. 1 . PCs were calculated utilizing all the Finnish data with the princomp-function of R. The first 22 components explained >95% of the variation, of which the six first components explained >80% of the variation in the data set ( Supplementary Data ). The remaining 16 components explained only <2% of variation each. On the basis of PCs, the multiple testing corrected significance level was set to P <0.05/22 components = P <0.0023. The PCs did not follow clear physiological categories. Heat map of metabolite levels To visualize the change in metabolite concentrations by age in FINRISK-97, the mean of the standardized metabolite level per 1-year age group (age, age+1) was plotted for each metabolite and sex. Metabolite standardization and plotting were performed separately for males and females. In the standardization, the mean of under 35-year olds was used as reference instead of the mean of all observations to account for the dissimilarities in age distributions between the sexes (mean age 45.1 in FINRISK-97 females and 48.8 in males) and to compare against values of ‘metabolically healthy’ individuals. The change in colour represents, thus, the divergence in units of s.d.’s from the mean of the metabolite levels of 24–35-year olds. Clear individual metabolite outlier values (from 13 subjects in FINRISK-97) were removed before metabolite standardization to prevent individual age groups from standing out due to outliers. The heat maps were plotted in a similar manner in the Estonian EGCUT cohort with 24–35 year olds as the reference age group. Age–sex interaction and splines Age–sex interactions were assessed with an age × sex interaction term in a random effects meta-analysis (rma.uni-function in metafor package of R, mean I 2 =35.2) using a linear regression model, adjusted further for BMI, daily smoking status (as a dichotomous variable), and fasting time (hours) before sampling ([metabolite~age × sex+BMI+daily smoking+fasting time). Random effects model was employed in all analyses because of differences in the characteristics of cohorts used, as seen in Table 1 , and for better comparison between different metabolites. Men and women aged 40–55 years, that is, the age overlapping the menopausal transition period, from three Finnish cohorts (FINRISK-97, DILGOM and Health2000, comprising participants in the selected age group, n =3,478) were included in the analysis. Metabolites were normalized separately by rank-based inverse normal transformation within each cohort. Natural cubic splines were constructed of all the Finnish participants with the ns-function of the splines package of R. Splines are based on the s.d.-normalized score of the metabolite concentrations with knots placed every 5 years of age. Menopause analyses Menopausal effects were explored with random effects meta-analysis using the restricted maximum-likelihood estimator approach [68] , [69] (rma.uni-function with method=’REML’ in metafor package of R) utilizing [70] a linear regression model (metabolite~menopause status+age+BMI+daily smoking+fasting time). The FINRISK-97 and the DILGOM cohorts were additionally adjusted for the geographical eastern-western status. Menopause status was assessed as a dichotomous variable. To achieve normality, rank-based inverse normal transformation was applied to the metabolite concentrations, to attain the means of zero and s.d.’s of one. The first phase comprised 10,083 women from Finland and Estonia (age range 21–75 years, mean I 2 =73.5). The analysis was then further targeted to those women in the menopausal transition window (aged 40–55 years, n =3,204, mean I 2 =27.2). The I 2 figures are from meta-analysis performed as stated above. How to cite this article: Auro, K. et al. A metabolic view on menopause and ageing. Nat. Commun. 5:4708 doi: 10.1038/ncomms5708 (2014).